Experimental realization of quantum zeno dynamics It is generally impossible to probe a quantum system without disturbing it. However, it is possible to exploit the back action of quantum measurements and strong couplings to tailor and protect the coherent evolution of a quantum system. This is a profound and counterintuitive phenomenon known as quantum Zeno dynamics. Here we demonstrate quantum Zeno dynamics with a rubidium Bose–Einstein condensate in a five-level Hilbert space. We harness measurements and strong couplings to dynamically disconnect different groups of quantum states and constrain the atoms to coherently evolve inside a two-level subregion. In parallel to the foundational importance due to the realization of a dynamical superselection rule and the theory of quantum measurements, this is an important step forward in protecting and controlling quantum dynamics and, broadly speaking, quantum information processing. Back action is a concept that lies at the very heart of quantum mechanics. In contrast to classical mechanics, it is impossible to probe a quantum system without disturbing it (unless the system is in an eigenstate of the observable). Yet, quantum mechanics allows the exploitation of back actions to drive the dynamics along different quantum paths. As first noticed by von Neumann [1] , a given quantum state can indeed be guided into any other state by tailoring a specific sequence of measurements. When the measurements lead back to the initial state and are frequent enough [2] , the back action freezes out the dynamics: a prominent example of measurement-induced disturbance that later took the name of the quantum Zeno effect (QZE) [3] . The QZE was first experimentally proven in a closed system to significantly slow down Rabi-driven oscillations between two levels [4] . In open systems, the Zeno effect as well as an acceleration due to an anti-Zeno effect [5] , [6] were first demonstrated in ref. 7 . Notice that both effects can also influence thermalization [8] . A general approach for the control of quantum behavior by coupling to the continuum was presented in ref. 6 . However, quantum Zeno does not necessarily imply a freeze-out. Quite to the contrary, back actions can also be exploited to preserve a coherent dynamics in a subspace of the Hilbert space and to forbid transitions among engineered boundaries. This phenomenon is known as quantum Zeno dynamics (QZD) and has been predicted in ref. 9 . A possible implementation of QZD with atoms in optical cavities has been theoretically investigated in ref. 10 . Here we experimentally realize QZD in a five-level Hilbert space describing a Bose–Einstein condensate (BEC) of 87 Rb atoms in a magnetic microtrap. In particular, by means of engineered strong couplings and controlled measurements, different regions of the Hilbert space can be dynamically disconnected, that is, the transfer of a physical state from one of this region to another is dynamically forbidden. This corresponds to projecting the full Hamiltonian into an effective one, with the latter involving only part of the Hilbert space. Furthermore, the distinctive controllability of our physical system allows us to apply four different coupling protocols and to show how to confine 87 Rb atoms in a two-level subregion, where they evolve coherently. This is also tested via Ramsey interferometry and successfully compared with a simple theoretical model. Finally, we demonstrate that the four different coupling protocols lead to the same QZD evolution. This constitutes also the first experimental verification of the theoretical prediction [11] that QZD can be equivalently attained (asymptotically) by frequent projective measurements, strong continuous coupling and fast unitary kicks. Experimental setup In this study we present experimental results obtained on a rubidium ( 87 Rb) BEC evolving in a five-level Hilbert space given by the five spin orientations of the F =2 hyperfine ground state (see Fig. 1 ). We use a time sequence of pulses to perform a state-selective negative measurement, namely a measurement of the absence of population from one particular level of the system. This dynamically decouples the Hilbert space in two-level subregions. The atoms are found to oscillate coherently between the states | F , m F ›=|2, 2›≡|↑› and |2, 1›≡|↓› without leaking out to the other available states. The same results have been obtained in the absence of measurements by exploiting unitary couplings, both constant and pulsed in time. This proves the prediction [11] that measurements are not a crucial ingredient for attaining QZD. We further prove via Ramsey interferometry that the strong back actions preserve, rather than destroy, the coherence of the atomic two-level superposition. 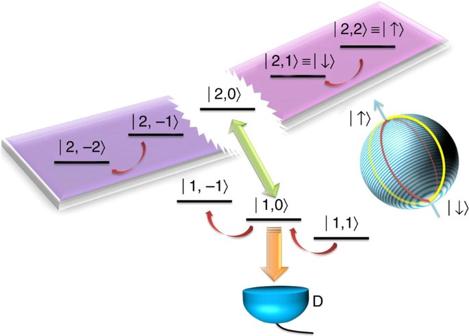Figure 1: Representation of our QZD scheme. Shown is the level structure of the87Rb atom cloud that is initially in the |F,mF›=|2,2› state. The levels of the protected two-level subspace are |2, 2› and |2, 1›, denoted as |↑› and |↓›, respectively. An applied RF field at 2.171 MHz couples neighbouringmFstates (thin, red arrows), a laser-induced Raman transition couples the |2, 0› and |1, 0› states (thick, green arrow). The hyperfine splitting between theF=2 andF=1 manifolds is ~6.834 GHz. An additional laser field connects theF=1 states to an external level (thick, orange arrow) and induces dissipation by spontaneous decay (lifetime 6 ns). This corresponds to the detection D. Rabi oscillations (around anxaxis) and Ramsey rotations (yaxis) of the protected two-level subspace, discussed later in the text, are indicated on the Bloch sphere13. Figure 1: Representation of our QZD scheme. Shown is the level structure of the 87 Rb atom cloud that is initially in the | F , m F ›=|2,2› state. The levels of the protected two-level subspace are |2, 2› and |2, 1›, denoted as |↑› and |↓›, respectively. An applied RF field at 2.171 MHz couples neighbouring m F states (thin, red arrows), a laser-induced Raman transition couples the |2, 0› and |1, 0› states (thick, green arrow). The hyperfine splitting between the F =2 and F =1 manifolds is ~6.834 GHz. An additional laser field connects the F =1 states to an external level (thick, orange arrow) and induces dissipation by spontaneous decay (lifetime 6 ns). This corresponds to the detection D. Rabi oscillations (around an x axis) and Ramsey rotations ( y axis) of the protected two-level subspace, discussed later in the text, are indicated on the Bloch sphere [13] . Full size image The initial state of all the experiments presented in the following is a cloud of 87 Rb atoms in the |↑› state Bose condensed in a magnetic trap. After creation of the condensate (see Methods for more details on the experimental procedure), the atoms are released from the trap. A homogeneous magnetic bias field defines the quantization axis of the system and lifts the degeneracy of the states. We then shine a radio frequency (RF) field resonantly coupling neighbouring m F states in the F =2 manifold. Under the effect of the RF field, the system evolves according to the Hamiltonian where the basis is chosen to start from m F =+2. It is obtained by applying angular-momentum algebra and the rotating-wave approximation [12] . Here and in the following, we set ℏ =1 and express all energies in angular frequencies. The Rabi frequency Ω is proportional to the RF field intensity. We choose Ω =2 π × 15 kHz. As a result of this interaction, the atomic population cycles periodically between all the five sublevels of the F =2 manifold as shown in Fig. 2a . 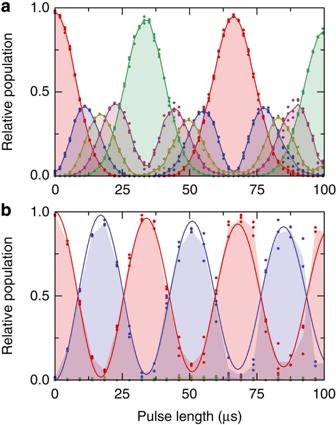Figure 2:Rabi oscillations observed in theF=2 manifold. (a) With only the RF field applied. Experimental data are represented by dots. As there is not sufficient data for statistically significant error bars, we instead report all the data from three runs of the experiment. The shaded areas correspond to their average values, whereas the lines are the model predictions of equation (1). The relative populations (mF=+2: red; +1: blue; 0: yellow; −1: violet; −2: green) are reported as function of the RF pulse length. The observed oscillations involve all five states. (b) With RF field plus constant Raman beams of coupling strength 2π× 200 kHz applied. The figure is organized as ina, but for the solid lines that here represent the solution of equation (3). The populations oscillate between the |2, 2›≡|↑› (red) and |2, 1›≡|↓› (blue) states. The observed oscillations decay, because at finite Raman powers the atoms eventually leak out of the protected subspace and into the (here unobserved)F=1 hyperfine states. Figure 2: Rabi oscillations observed in the F =2 manifold. ( a ) With only the RF field applied. Experimental data are represented by dots. As there is not sufficient data for statistically significant error bars, we instead report all the data from three runs of the experiment. The shaded areas correspond to their average values, whereas the lines are the model predictions of equation (1). The relative populations ( m F =+2: red; +1: blue; 0: yellow; −1: violet; −2: green) are reported as function of the RF pulse length. The observed oscillations involve all five states. ( b ) With RF field plus constant Raman beams of coupling strength 2 π × 200 kHz applied. The figure is organized as in a , but for the solid lines that here represent the solution of equation (3). The populations oscillate between the |2, 2›≡|↑› (red) and |2, 1›≡|↓› (blue) states. The observed oscillations decay, because at finite Raman powers the atoms eventually leak out of the protected subspace and into the (here unobserved) F =1 hyperfine states. Full size image State-selective measurements We implement a state-selective measurement as a two-step process: a full population transfer from |2, 0› to |1, 0› is followed by a population measurement of the latter. Technically speaking, the first two laser beams (‘Raman beams’) induce a Raman transition between |2, 0› and |1, 0›. We then illuminate the BEC with a laser beam (‘Dissipative Light’) resonant with the F =1→ F ′=2 transition to the 5 P 3/2 excited state from which atoms will decay outside the BEC. During the decay, a photon is emitted [4] . This process is commonly considered a measurement even if the emitted photon is not detected. Note that this radiation will only affect atoms in the F =1 state, that is, atoms that were originally in |2, 0›. To show which ingredients are really mandatory to achieve QZD, we implement four different experimental protocols: in the first one, we realize a series of discrete measurements by a periodic application of our state-selective measurement scheme. In the second protocol, we apply continuously both the Raman beams and the Dissipative Light, and we perform a continuous measurement. In the third and fourth protocols, no Dissipative Light is used and the dynamics is unitary. In the third experiment, unitary kicks are realized by a sequence of π -pulses of the Raman beams. In the fourth protocol, we implement a continuous coupling scheme and the Raman beams are kept on continuously. See Methods for details on the parameters chosen in each case. In all these experiments, by means of the Raman beams we are effectively observing the absence of any population in the |2, 0› state. In the language of QZD [11] , this accounts to projecting our Hamiltonian equation (1) into an effective one, H ′= PHP , where P is the projector on the subspace spanned by all sublevels except the observed one, |2, 0›. As we start with all the population in state |↑›, we expect the evolution to be restricted to the two states |↑› and |↓›. A typical result obtained with our fourth protocol (continuous unitary coupling) is reported in Fig. 2b . In contrast to the case of purely RF-induced oscillations ( Fig. 2a ), the population now oscillates between the first two sublevels only (rotations around x axis in the Bloch sphere [13] in Fig. 1 ), with nearly negligible decay toward the other levels. This is the hallmark of QZD. Experimental results A comparison of the results obtained with the four different protocols is given in Fig. 3 . For the chosen parameters, we observe a similar population dynamics. This is in close agreement with the prediction [11] that frequent projective measurements, strong continuous coupling or fast unitary kicks should all asymptotically lead to a confined dynamics according to equation (2). As indicated by our experimental results, the degree of confinement can be strong and comparable (within the experimental error bars) even with finite measurement rates and coupling strengths. This freedom is important with respect to future applications of QZD. 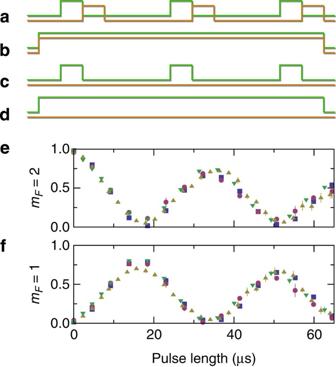Figure 3: Comparison of four different protocols to induce QZD. Shown is a comparison between RF-induced Rabi oscillations for all four experimental protocols: (a) discrete measurements (green down triangles), (b) continuous measurements (violet circles), (c) unitary kicks (yellow up triangles) and (d) continuous unitary coupling (blue squares). See Methods section for details on the chosen parameters. (e,f) The relative populations in themF=2 andmF=1 states, respectively, as a function of total RF pulse length. We report the average populations with error bars (mostly comparable to the data symbol size) indicating the spread of the data. The lower four sets of lines illustrate the time sequences of the four protocols. The Raman beams are in green, the Dissipative Light is in orange. The horizontal time axis is not to scale. Figure 3: Comparison of four different protocols to induce QZD. Shown is a comparison between RF-induced Rabi oscillations for all four experimental protocols: ( a ) discrete measurements (green down triangles), ( b ) continuous measurements (violet circles), ( c ) unitary kicks (yellow up triangles) and ( d ) continuous unitary coupling (blue squares). See Methods section for details on the chosen parameters. ( e , f ) The relative populations in the m F =2 and m F =1 states, respectively, as a function of total RF pulse length. We report the average populations with error bars (mostly comparable to the data symbol size) indicating the spread of the data. The lower four sets of lines illustrate the time sequences of the four protocols. The Raman beams are in green, the Dissipative Light is in orange. The horizontal time axis is not to scale. Full size image To quantify the coherence of the dynamically created two-level system, we describe the observed oscillations obtained with our fourth protocol with an effective two-state model (see Methods). We introduce phenomenologically the rate Γ loss to account for losses from state |↓› to external states and γ deph to account for the loss of coherence between the states |↑› and |↓›. These two terms have different physical origin. The rate Γ loss arises from the imperfect protection of the Zeno subspace due to our finite coupling strength [14] . The dephasing rate γ deph is originated in our experiment by the presence of high-frequency noise on the magnetic bias field and the RF signal, and by off-resonant scattering of photons from the Raman beams. This model is valid only for short evolution times. Because of the finite size of our Hilbert space and the finite coupling strength, the population can come back to the initial state, |↑›. This means that for long times we experience a revival of population into the Zeno (partially)-protected subspace. Therefore, we apply our two-level model only for times up to 100 μs, where the population revival is still not affecting the observed dynamics. In Fig. 2b , we included a fit of our model to the experimental data of the population dynamics of the states |↑› and |↓›. From the fit, we extract the values γ deph =2 π × 0.3 −0.2 +0.3 kHz and Γ loss =2 π × 0.02 −0.02 +0.12 kHz, corresponding to a lifetime of the particles in the subspace of 50 ms. In the upper panel of Fig. 4 , we report the dephasing times, 2 π / γ deph , obtained by a scan of the Raman couplings in the range from 2 π × 100 to 2 π × 225 kHz. Only a weak dependence of the dephasing rate on the Raman coupling is observed. 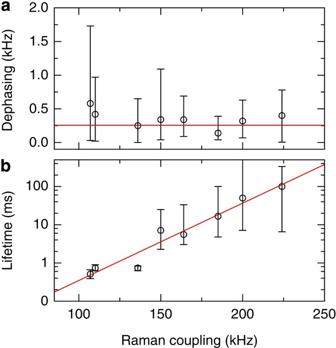Figure 4: Dephasing and lifetimes in a protected subspace. The dephasing rates (a) and lifetimes (b) of the atom population in the protected subspace under constant Raman beams illumination are reported. The factor 2πin the coupling frequencies is suppressed. The RF-induced Rabi coupling is constant at 2π× 15 kHz. The data (points) are well fitted (red lines) by a constant dephasing rate and by an exponentially increasing lifetime, respectively. The error bars indicate the uncertainty in the parameter estimation (see Methods for details). The dephasing rates display only a weak dependence on the Raman coupling strength. The lifetimes are observed to increase hundredfold. Figure 4: Dephasing and lifetimes in a protected subspace. The dephasing rates ( a ) and lifetimes ( b ) of the atom population in the protected subspace under constant Raman beams illumination are reported. The factor 2 π in the coupling frequencies is suppressed. The RF-induced Rabi coupling is constant at 2 π × 15 kHz. The data (points) are well fitted (red lines) by a constant dephasing rate and by an exponentially increasing lifetime, respectively. The error bars indicate the uncertainty in the parameter estimation (see Methods for details). The dephasing rates display only a weak dependence on the Raman coupling strength. The lifetimes are observed to increase hundredfold. Full size image A complete suppression of a leakage of atoms out of the two-level subspace is only expected at infinite Raman coupling strength where the projector P of equation (2) would be exactly realized. In Fig. 4 (lower panel), we report the lifetimes 2 π /Γ loss obtained for different settings of the Raman coupling strength. We observe a crossover from a full five-level dynamics at 100 kHz to a nearly pure two-level dynamics above 200 kHz. In this range, the lifetime increases 100-fold at an exponential rate of about 0.05 kHz −1 . To further investigate the coherence of the dynamics in the two-level subspace, we realized a Ramsey interferometric scheme within the two-level subspace (corresponding to rotations around the y axis in the Bloch sphere in Fig. 1 ). In the presence of constant Raman beams, two RF pulses are sent onto the atoms separated by a variable delay time T . Each RF pulse encompasses a π /2 area such that the first pulse evenly populates the two states of our subspace. Note that this is impossible in the absence of the Raman beams as was already observed in ref. 15 . The populations after the second pulse are then recorded as a function of T . An oscillatory population distribution between the two sublevels is expected if and only if there is coherence between both states [16] . We report our experimental findings in Fig. 5 . The populations show clear oscillations with fringe contrast close to unity over the whole observed pulse delay range T . Only a small damping of the oscillations is perceivable. This concludingly confirms that QZD preserves the coherence of the dynamics in protected subspaces. 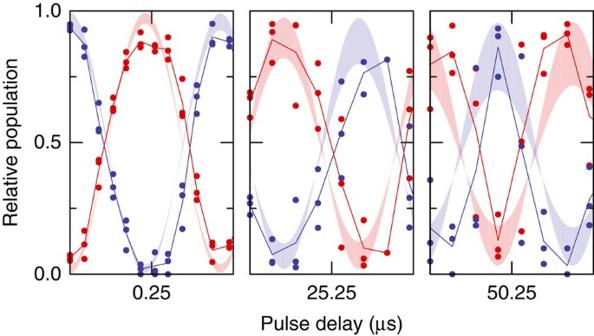Figure 5: Demonstration of coherent dynamics. A Ramsey scheme experiment reveals interference fringes as function of the delay timeTbetween the two RF pulses. For better resolution, we show the data obtained only in three ranges ofT. Each window has a temporal width of 0.5 μs. Reported are the populations of the |↓› (red) and |↑› (blue) states. Shown are the raw data (points, three measurements per delay time), their mean values (connected straight lines) and the model prediction (shaded areas) with the corresponding parameters taken fromFig. 4. The Raman beams induced a coupling strength of 2π× 140 kHz. In the observed pulse delay range, only a small loss of fringe contrast is noted. Figure 5: Demonstration of coherent dynamics. A Ramsey scheme experiment reveals interference fringes as function of the delay time T between the two RF pulses. For better resolution, we show the data obtained only in three ranges of T . Each window has a temporal width of 0.5 μs. Reported are the populations of the |↓› (red) and |↑› (blue) states. Shown are the raw data (points, three measurements per delay time), their mean values (connected straight lines) and the model prediction (shaded areas) with the corresponding parameters taken from Fig. 4 . The Raman beams induced a coupling strength of 2 π × 140 kHz. In the observed pulse delay range, only a small loss of fringe contrast is noted. Full size image We have demonstrated that measurements and strong couplings can be tailored to create disjoint Hilbert subspaces. We have shown that a two-level system initially localized in one of this subspaces will evolve coherently without leaking probability to neighbouring Hilbert subspaces. This realizes a dynamical superselection rule, which, in analogy to the ‘W3’ superselection rule for charge [17] , imposes that if two initial states are separated in different regions of the Hilbert space, the separation will persist at all times. A general crucial problem of quantum information is to protect experimental protocols from decoherence and probability leakage. A strategy discussed in the literature is to encode the information on a part of the overall Hilbert space where noise cancels out. The existence of such decoherence-free subspaces was demonstrated in refs 18 , 19 . Moreover, strategies for bath-optimized protection of quantum information were discussed [20] . Here we provide the proof-of-principle of an alternative noise-protection scheme, which is realized via four different protocols. The idea is to dynamically exploit QZD to drive the dynamics inside a designed region of the full space of accessible states and preserve quantum coherence against any leakage to the environment. It is noteworthy that, although in a different context and perspective, a broad variety of pulse control techniques have been developed and used in NMR quantum computation to suppress decoherence and confine the dynamics in subsystems [21] , [22] and, very recently, also for nitrogen-vacancy centres in diamonds [23] . A future exploration of QZD in our five-level system will be the realization of a controllable two-qubit gate, where strong couplings are exploited to protect the two different qubits and tailor their interaction. In view of possible applications, one could implement all sources necessary for our schemes in a single integrated device by replacing the Raman beams with microwave radiation. The possibility of engineering the coupling of the system to the environment for quantum state preparation and quantum computation is of particular relevance as shown theoretically in refs 24 , 25 , 26 , 27 . Our approach can be explored in other physical systems, such as quantum cavities or trapped ions, realizing multilevel subspaces (qudits) or continuous-variable ones. Therefore, our results open up the way to the control of quantum information systems in the broader sense of QZD. Creation of the 87 Rb BEC We produce a BEC of 87 Rb atoms in a magnetic microtrap realized with an atom chip (see upper part of Fig. 6 ). The apparatus consists of a single cell only, for both initial atom trapping and BEC creation. The main component of the magnetic trap consists of a Z -shaped wire on the atom chip with just 125 μm diameter that hosts a current of 1.8 A. The magnetic trap is completed by an external pair of Helmholtz coils. The loading procedure starts by emission of hot Rb atoms into the vacuum cell by means of a pulsed Rb dispenser. The atoms are then laser cooled in a magneto-optical trap and transferred to the chip trap using an ancillary magnetic trap realized by sending a current of 25 A through a wire (1 mm diameter) placed behind the chip (not visible in Fig. 6 ). BEC is reached in 8 s by forced evaporative cooling, ramping down the frequency of an RF field. The RF fields for evaporation and manipulation of the Zeeman states are produced by two further conductors also integrated on the atom chip. The BEC has typically 8 × 10 4 atoms, a critical temperature of 0.5 μK and is at 300 μm from the chip surface. The trap has a longitudinal frequency of 46 Hz and the radial trapping frequency is 950 Hz. Substantial heating of the atom chip during the chip-loading phase and the need for pumping out all the polluting gas emitted by the dispenser impose a 15-s recovery time. 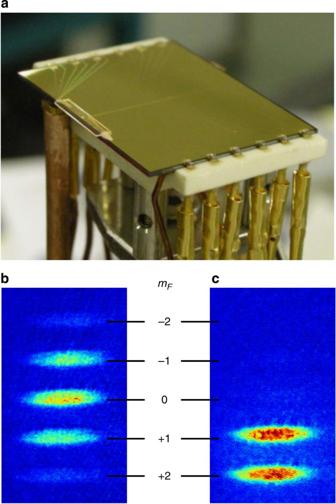Figure 6: Rb BEC on an atom chip. (a) Picture of the atom chip before it was installed inside the vacuum system. Visible is the chip (23 mm × 30 mm) with its reflective, golden surface. On its left, an embedded photonic structure (not used in the present experiment) is visible. Two rows of wires interface the chip structures with the experiment control. In the final setup, the chip is mounted upside down. (b,c) Absorption images taken 24 ms after release from the magnetic trap. Inbis shown the population distribution after an RFπ/2 pulse in the absence of the Raman beams. The population is centred around |2, 0›. (c) The situation with constant Raman beams. An appropriate RFπ/2 pulse now even populates the |↑› and |↓› states. This configuration is used to initialize the Ramsey interferometer in the protected subspace. Thus, a complete experimental cycle has a duration of 23 s. Figure 6: Rb BEC on an atom chip. ( a ) Picture of the atom chip before it was installed inside the vacuum system. Visible is the chip (23 mm × 30 mm) with its reflective, golden surface. On its left, an embedded photonic structure (not used in the present experiment) is visible. Two rows of wires interface the chip structures with the experiment control. In the final setup, the chip is mounted upside down. ( b , c ) Absorption images taken 24 ms after release from the magnetic trap. In b is shown the population distribution after an RF π /2 pulse in the absence of the Raman beams. The population is centred around |2, 0›. ( c ) The situation with constant Raman beams. An appropriate RF π /2 pulse now even populates the |↑› and |↓› states. This configuration is used to initialize the Ramsey interferometer in the protected subspace. Full size image All subsequent manipulations are made 0.7 ms after turning off the magnetic trap to guarantee bias field homogeneity (at 3.1 Gauss, corresponding to an energy splitting of the Zeeman states of about 2.2 MHz) and strongly reduce the effects of atomic collisions. To drive the Raman transition, we derived from a diode laser source two coherent beams, one of them passing an electro-optic modulator plus Fabry–Pérot cavity combination to shift its frequency by 6.834 GHz. The laser beams with mutually perpendicular linear polarizations are red detuned by about 18 and 25 GHz from the nearest resonance of the D2 line at 780 nm. The beams have their waist of ~70 μm on the atomic sample and are propagating collinearly in the direction parallel to the applied bias field. As the Landé factors of the two hyperfine states have opposite signs (cf. Fig. 1 of the main text), in the presence of the bias magnetic field, the two laser beams can be resonant only with a single pair of levels at a time. We choose the frequency difference such that the connected levels are |2, 0› and |1, 0›. To maximize the transfer efficiency, the beam intensities are chosen to be equal. We can induce oscillations with frequencies up to 400 kHz. Off-resonant scattering from the excited states damps these oscillations in around 50 μs. The illumination with Dissipative Light can remove all atoms from the F =1 state in 0.6 μs. Note that the emission of a spontaneous photon is enough to kick the atoms out of the BEC. Therefore, this interaction is, for our purpose, completely destructive. To record the number of atoms in each of the m F states of the F =2 hyperfine state, we apply a Stern–Gerlach method. After 1 ms of free expansion in addition to the homogeneous bias field, an inhomogeneous magnetic field is applied along the quantization axis for 10 ms. This causes the different m F states to spatially separate. After a time of 23 ms of expansion, a standard absorption imaging sequence is executed (see Fig. 6 , lower part). By performing interleaved control measurements (by not turning on the RF field), we distinguish the fraction of atoms lost from the F =2 manifold due to leakage out of the protected two-level system from atoms lost due to residual scattering of the Raman and Dissipative Light beams. Losses due to collisional heating induced by the Dissipative Light are up to ~50% during the experimental sequence. The data are corrected not to include losses due to scattering. Density matrix two-level model The two-level model expressed in terms of the density matrix ρ is where ρ ii , ( i = α , β ) is the population of the levels m F =2 and m F =1, respectively, and ρ αβ is their coherence. The error intervals of the fit are taken as the range where the squared sum of the fit residuals worsens by 10% under variation of one parameter only. QZD via four different protocols To induce QZD, four different protocols were exploited. Here we report details on the experimental parameters for each protocol. In the first protocol, discrete measurements, a sequence of double pulses is applied to the atoms. We first apply a 0.8-μs π -pulse (that is, a pulse that transfers all the atoms that might be present in the |2, 0› state to the |1, 0› state) with the Raman beams. Immediately after this pulse, we apply for 0.6 μs the Dissipative Light. As a result of this sequence, any atom that would have been initially present in |2, 0› would be detected. We repeat this sequence every 2.2 μs. For the second protocol, continuous measurements, we apply both the Raman beams and the Dissipative Light continuously. The intensities are chosen such as to obtain a Raman-induced coupling of 2 π × 250 kHz and a dissipative loss rate of 2 π × 450 kHz. The intensity of the Dissipative Light was chosen such as to induce a loss rate only slightly above the Raman coupling rate. This was done to avoid blocking the Raman transition by a Dissipative Light-induced QZE, while still implementing an effective measurement scheme. Our third protocol, unitary kicks, consists of sending a sequence of isolated pulses onto the atoms. The Raman beams π -pulses have a duration of 0.7 μs and are repeated every 2.2 μs. The fourth protocol, continuous unitary coupling, relies on the sole usage of the Raman beams. They are tuned to a coupling strength of 2 π × 136 kHz. With the chosen parameters, the lifetimes 2 π /Γ loss are observed to be in the range 0.7–1.0 μs. The decoherence rates γ deph are found to lie between 2 π × 0.3 and 2 π × 0.8 kHz. How to cite this article: Schäfer, F. et al. Experimental realization of quantum zeno dynamics. Nat. Commun. 5:3194 doi: 10.1038/ncomms4194 (2014).